The microbiome of New World vultures Vultures are scavengers that fill a key ecosystem niche, in which they have evolved a remarkable tolerance to bacterial toxins in decaying meat. Here we report the first deep metagenomic analysis of the vulture microbiome. Through face and gut comparisons of 50 vultures representing two species, we demonstrate a remarkably conserved low diversity of gut microbial flora. The gut samples contained an average of 76 operational taxonomic units (OTUs) per specimen, compared with 528 OTUs on the facial skin. Clostridia and Fusobacteria, widely pathogenic to other vertebrates, dominate the vulture’s gut microbiota. We reveal a likely faecal–oral–gut route for their origin. DNA of prey species detectable on facial swabs was completely degraded in the gut samples from most vultures, suggesting that the gastrointestinal tracts of vultures are extremely selective. Our findings show a strong adaption of vultures and their bacteria to their food source, exemplifying a specialized host–microbial alliance. The microbiota of vertebrates rapidly begin to decompose their hosts after death [1] . During the subsequent breakdown of tissue, these microorganisms excrete toxic metabolites, rapidly rendering the carcass a hazardous food source for most carnivorous and omnivorous animals [2] . Some scavengers such as vultures, however, are able to consume carrion without suffering any apparent ill-effects. Indeed, vultures may have to wait for decay to occur before they are able to scavenge carcasses with tough skins, thus substantially increasing the risk of exposure to toxins [3] . Furthermore, to obtain access to the inside of such carcasses, they often insert their heads directly in the body cavities of decaying prey, thereby exposing their head and neck to pathogenic bacteria [3] . Although the majority of the ingested bacteria will not survive the acidic gastric passage before hindgut colonization, toxins such as botulinum survive the passage into the hindgut, possibly seriously compromising the health of the consumer [4] . Furthermore the pioneering feeding experiments of Houston and Cooper revealed that spore forming pathogens such as Bacillus anthracis can be recovered from vulture faeces [5] . To investigate how vultures are able to tolerate this challenging dietary niche, here we characterize the functional microbiome of the facial skin and the hindgut (large intestine) of the two most widespread species of vultures in the New World ( Coragyps atratus (black vulture) n= 26; Cathartes aura (turkey vulture) n= 24; both collected in Nashville, USA). We show that the acidic gastrointestinal tract of vultures is a strong filter of the microbiota ingested from decaying carcasses resulting in a significantly less diverse hindgut flora dominated by Clostridia and Fusobacteria, which are pathogenic to most vertebrates. Facial DNA reveals prey composition We initially investigated whether an individual’s diet, as assayed from facial swabs, influenced the bacterial composition of the vulture’s face and hindgut. This was done via PCR amplification and deep sequencing of a mammalian-generic mitochondrial 16S rRNA gene. Amplification of potentially contaminating human DNA was reduced by the addition of blocker oligos during PCR. Although these primers have been successfully used in other dietary DNA studies [6] , [7] , [8] , we detected mammalian amplicons in only four (8%) of the vulture hindgut samples (all turkey vultures). In contrast, mammalian DNA was readily amplified from most facial swabs (~90%), representing nine mammalian families ( Bovidae , Canidae , Cervidae , Didelphidae , Equidae , Leporidae , Mephitidae , Procyonidae , Suidae ). 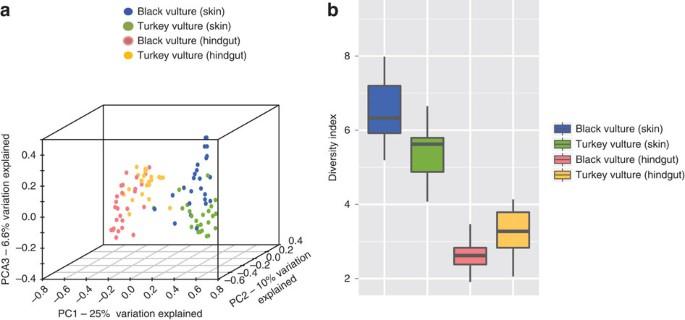Figure 1: Facial skin and hindgut exhibit largely different microbial communities. (a) Microbial clustering on the basis of Bray–Curtis dissimilarity matrix (visualized by principal coordinate analysis). Facial skin and hindgut communities exhibited minor overlap (ANOSIM;R=0.744,P=0.001). Hindgut (ANOSIM,R=0.333,P=0.001) and skin (ANOSIM,R=0.321,P=0.001) communities showed minor clustering within vulture species. (b) Variation in diversity (Shannon index) in facial skin and hindgut. The hindgut community was significantly less diverse than the facial community (Wilcoxon Rank-Sum test,P≪0.001). The facial communities of the black vulture were more diverse than those of the turkey vulture whereas the hindgut samples displayed the opposite pattern (Wilcoxon Rank-Sum test,P≪0.01). There were no differences between male and female vultures in the clustering (not shown) of hindgut (ANOSIM,R=0.063,P>0.05) or facial (ANOSIM,R=0.025,P>0.05) communities. The majority of mammalian families were observed in both the vulture species ( Supplementary Table 1 ). Despite the use of human-specific blocking primers, human DNA was recovered from one turkey vulture facial swab and hindgut sample, most likely a laboratory contaminant but possibly from ingested sewage. The difference in mammalian DNA on the facial swabs and from the hindgut reflects the significant breakdown of dietary DNA in the vulture gastrointestinal tract pointing to extraordinarily harsh chemical conditions that may be an adaptation to the consumption of toxic carrion. Therefore the microbial flora colonizing the vulture gastrointestinal tract has adapted to survive these harsh conditions. To investigate the microbiota of the scavengers, we PCR amplified and deep sequenced a microbial ribosomal phylogenetic marker from each DNA extraction. Microbial communities assemble similarly in both vulture species A clear distinction was observed between the microbial communities ( Fig. 1a ) of the facial skin (black vulture, n =26, 4,221–8,661 reads per animal, ; turkey vulture, n =24, 3,104–8,770 reads per animal, ) and hindgut samples (black vulture, n =26, 4,868–10,241 reads per animal, ; turkey vulture, n =23, 3,376–10,825 reads per animal, ). The facial microbial community was significantly more diverse than that of the hindgut ( Fig. 1b ), inconsistent with previous observations from other vertebrates such as humans [9] . The skin and hindgut microbiota of turkey and black vultures largely overlapped, consistent with the observation that both species routinely feed on the same prey species and often at the same carcasses ( Fig. 1a ). Figure 1: Facial skin and hindgut exhibit largely different microbial communities. ( a ) Microbial clustering on the basis of Bray–Curtis dissimilarity matrix (visualized by principal coordinate analysis). Facial skin and hindgut communities exhibited minor overlap (ANOSIM; R =0.744, P =0.001). Hindgut (ANOSIM, R =0.333, P =0.001) and skin (ANOSIM, R =0.321, P =0.001) communities showed minor clustering within vulture species. ( b ) Variation in diversity (Shannon index) in facial skin and hindgut. The hindgut community was significantly less diverse than the facial community (Wilcoxon Rank-Sum test, P ≪ 0.001). The facial communities of the black vulture were more diverse than those of the turkey vulture whereas the hindgut samples displayed the opposite pattern (Wilcoxon Rank-Sum test, P ≪ 0.01). There were no differences between male and female vultures in the clustering (not shown) of hindgut (ANOSIM, R =0.063, P >0.05) or facial (ANOSIM, R =0.025, P >0.05) communities. Full size image Clostrida and Fusobacteria prevail in the vulture gut Given the challenge of penetrating the hide of large mammals, vultures often enter large carcasses through natural orifices, in particular the anus [5] . This increases the likelihood of ingesting anaerobic faecal bacteria such as Clostridia and Fusobacteria [10] . Indeed, both bacterial groups were detected at high frequencies in the gut of both vulture species. The percentage of Clostridia sequence counts relative to total counts within the guts of individuals was largely similar in black vultures (min=26% and max=85%, ) and turkey vulture (min=26% and max=84%, ; Wilcoxon P >0.05). In contrast, percentages of Fusobacteria were significantly lower in the guts of black vultures (min=0.2% and max=54%, ) than in turkey vultures (min=2% and max=69%, ; Wilcoxon, P ≪ 0.05). There was no significant difference in the percentage of Clostridia on facial swabs from black vultures (min=7% and max=40%, ) and turkey vultures (min=8% and max=68%, ; Wilcoxon, P >0.05). Percentages of Fusobacteria were similar on the facial skin of black vultures (0% and max=31%, ) and turkey vultures (min=0.2% and max=23%, , Wilcoxon, P >0.05) as shown in Fig. 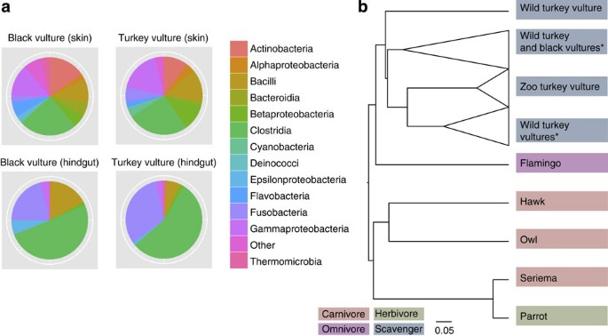Figure 2: Hindgut microbial flora of wild and zoo vultures is highly conserved. (a) Mean bacterial class distribution found on facial skin and in the hindgut of black and turkey vultures (see details inSupplementary Notes 1 and 2). (b) Comparison of microbial communities of zoo bird faeces and vulture hindguts (UPGMA tree based on Unifrac metric). The hawk, owl and vultures in the zoo received fresh meat. (Microbial composition of zoo bird faeces is given inSupplementary Note 3). *Clades collapsed. 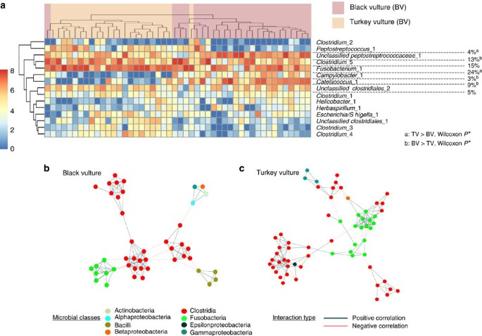Figure 3: Clostridia and Fusobacteria prevail in all hindgut samples and show negative co-occurrence patterns. (a) Heatmap of the log-transformed hindgut OTU abundance determined by 16S rRNA gene sequencing. Each displayed microbial OTU represents at least 2000 sequence observations across samples. The seven most frequent OTUs (---) accounted for more than 74% of all relative hindgut sequences generated (*P≪0.05,Supplementary Table 8). (b,c) Spearman co-occurence network cutoffρ=0.6,P≪0.05) generated from the OTU matrix. The displayed pairwise co-occurrences appeared in at least 50% of all hindgut vulture samples and are dominated by positive correlations. All observed negative correlations include either Clostridia or Fusobacteria. 2a and Supplementary Table 2 (see also observed genera in Supplementary Table 3 ). Although no comparable studies of facial skin microbiomes are available for comparison, these observations are unusual with regard to available vertebrate facial microbiomes, such as those of human (predominantly Actinobacteria), frogs (predominately Actinobacteria and Betaproteobacteria) and salamander (predominately Betaproteobacteria) [11] , [12] . Fusobacteria have not been reported on human skin. Clostridia on the other hand have been found to colonize parts of the human skin with lowered oxygen availability, for example the buttocks, but not the face [12] , [13] . Figure 2: Hindgut microbial flora of wild and zoo vultures is highly conserved. ( a ) Mean bacterial class distribution found on facial skin and in the hindgut of black and turkey vultures (see details in Supplementary Notes 1 and 2 ). ( b ) Comparison of microbial communities of zoo bird faeces and vulture hindguts (UPGMA tree based on Unifrac metric). The hawk, owl and vultures in the zoo received fresh meat. (Microbial composition of zoo bird faeces is given in Supplementary Note 3 ). *Clades collapsed. Full size image Oral–faecal route of gut bacteria The recovery of bacteria known to be linked to carcass degradation from vulture facial swabs renders it likely that at least part of the vulture facial microbiome, particularly Clostridia and Fusobacteria, are not necessarily skin colonizers, but originate from physical contact with food sources or soil clinging to the carcasses. There were 13,493 OTUs probably equivalent to bacterial species (black vulture, n =26; 346–1,534 OTUs per vulture; ; turkey vulture, n =24; 164–609 OTUs per vulture; ). Facial skin swabs contained significantly more microbes than hindgut samples (Welch’s t -test, P ≪ 0.001). We detected 1,551 OTUs in the hindgut samples (black vulture, n =26; 26–87 OTUs per vulture; ; turkey vulture n =23; 61–202 OTUs per vulture; ). Given that >85% of the microbial OTUs recovered at even sequencing depth (at 97% sequence similarity) were unique to the face, there appears to be a strong selection during the passage from the mouth to the gut. About half of the OTUs found in the hindgut occurred exclusively in the hindgut. However, OTUs common to facial skin and hindgut accounted for 98% of all hindgut sequences, including all bacterial specimens assigned to Clostridia and Fusobacteria. This provides strong evidence that majority of the hindgut microbes have the same origin as the facial bacteria. Furthermore, the average number of hindgut species for each vulture that were unique to that individual was only 10% (black vulture, , 3.5–36.7%; turkey vulture, , 1.5–26.6%; Welch’s t- test P ≪ 0.001; Supplementary Table 4 ) re-clustered at 96% sequence similarity for comparison with a previous study [14] . Thus ~90% of the vulture gut bacteria are shared between individuals. In comparison, the average unique OTU composition of the mammalian gut has been shown to be 56% (ref. 14 ). This observation demonstrates a stronger selection for the observed microbial community of vultures compared with mammals. Gut microbes are conserved between captive-bred and wild vultures To explore which components of the hindgut microbiome are unique to vultures, we generated additional avian metagenomic data using faecal samples obtained from several other species from a single location (Copenhagen Zoo). Samples included two captive-bred turkey vultures, three predatory species (red-tailed hawk ( Buteo jamaicensis ), African spotted owl ( Bubo africanus ), and red-legged seriema ( Cariama cristata )), a non-predatory Amazon parrot ( Amazona sp.) and the American flamingo ( Phoenicopterus ruber ). Recent studies of human gut dynamics have demonstrated that the gut microbiome can rapidly adjust to dietary modifications [15] . In addition, the gut microbiota of alligators has been observed to vary seasonally with diet [16] . It is notable that despite having similar diets in the zoo, the faecal microbiome of the zoo-kept turkey vultures was considerably different from those of the hawk and owl ( Fig. 2b , Supplementary Tables 5 and 6 ), but remarkably similar to the hindgut microbiome of the wild sampled vultures. This indicates that phylogenetic differences in the digestive physiology of vultures override the importance of diet in the assembly of the hindgut microbiota. Both Clostridia and Fusobacteria are common soil bacteria. However Clostridia species have been documented as the cause of severe food poisoning in both humans and chickens, and are responsible for periodic die-off of wild birds such as waterfowl and shorebirds [17] , [18] , [19] , [20] , [21] . Although the flesh-degrading Fusobacteria have been reported to colonize the hindgut of living omnivorous and carnivorous animals, in humans they do so at negligible abundances ( ≪ 1%) and have recently been shown to promote colon cancer (refs 14 , 22 , 23 ). Alligators, which scavenge carrion, exhibit similar frequencies of Clostridia and Fusobacteria as those observed in vultures, but vary over season [16] . However hyenas, mammalian carrion feeders, did not contain notable levels of Fusobacteria [14] . Thus, even though the vulture hindgut microbiota originated from the diet, we speculated that its composition is primarily shaped by the oral–gut passage and the hindgut properties. The frequency of Clostridia and Fusobacteria ( Fig. 3a ) in the hindgut raises the question of whether these bacteria simply outcompete other bacterial groups or if their presence is actually promoted for the physiological benefit of the vultures. The former option suggests that vultures are passive hosts that tolerate the bacteria and their toxins without receiving benefit, whereas the latter posits that the relationship is more mutualistic in that bacteria receive a predictable flow of protein-rich food in an anaerobic environment and the vultures obtain nutrients provided by bacterial degradation of carrion. Indeed we observed genes that encode tissue-degrading enzymes and toxins associated with Clostridium perfringens in the metagenome of the turkey vulture hindgut with shotgun sequencing ( Supplementary Table 7 ). Figure 3: Clostridia and Fusobacteria prevail in all hindgut samples and show negative co-occurrence patterns. ( a ) Heatmap of the log-transformed hindgut OTU abundance determined by 16S rRNA gene sequencing. Each displayed microbial OTU represents at least 2000 sequence observations across samples. The seven most frequent OTUs (---) accounted for more than 74% of all relative hindgut sequences generated (* P ≪ 0.05, Supplementary Table 8 ). ( b , c ) Spearman co-occurence network cutoff ρ =0.6, P ≪ 0.05) generated from the OTU matrix. The displayed pairwise co-occurrences appeared in at least 50% of all hindgut vulture samples and are dominated by positive correlations. All observed negative correlations include either Clostridia or Fusobacteria. Full size image Curiously, more than 90% of all microbial interactions in the hindguts of both vulture species ( Fig. 3b,c ) were of a positive nature. However, all negative co-occurrence interactions were assigned to either Clostridia and/or Fusobacteria, suggesting their competitive nature. Therefore, the most likely scenario is that Clostridia and Fusobacteria outcompete other bacterial groups in the anaerobic hindgut, and that vultures benefit from the bacterial breakdown of carrion while tolerating bacterial toxins. Some scavenging birds are known to harbour antibodies against toxins such as botulinum [24] and we speculate that vultures are unusually tolerant of toxins. In summary, our findings demonstrate that wild vultures host a similar but very unique gut microbiome that is dominated by two major groups of bacteria that likely originate from their food sources. To determine essential functions of vulture homeostasis contributed by the gut microbiota, germ-free vultures will need to be experimentally exposed to the microbes observed in this study, using mammalian investigations as a model [25] . The sampling of the wild vultures Coragyps atratus (Black vultures) were live-trapped at carcasses of road-killed deer at the same location over a period of several days. They were transported to a central facility within several hours of trapping and were then euthanized with CO 2 by USDA (United States Department of Agriculture) personnel under the authority of the US Fish & Wildlife Service. Vultures were necropsied and sampled within 30–45 min of death. Investigators were gloved, masked and gowned during the necropsies. Cathartes aura (Turkey vulture) were shot at roosts, bagged individually and quickly chilled to 2–4 °C. Vultures were then transported to the processing facility where they were refrigerated from 2 to 6 h before necropsy and sampling. Vulture trapping and euthanization procedures were approved by APHIS (Animal and Plant Health Inspection Service, USDA). Briefly, the hindgut (large intestine) samples were collected in a relatively sterile manner in a sheltered warehouse. Carcasses were opened ventrally from throat to vent to expose the entire gastrointestinal tract. We sampled sequentially from anterior to posterior. For all hindgut sampling, we isolated a 3–4 cm section of the large intestine about 2–3 cm above the cloaca with medical hemostats. A new sterile syringe was used for each sample. We injected 2–3 ml of sterile water through the wall of the hindgut with a sterile syringe (discarded after each aspiration), gently massaged the hemostat-blocked section of the hindgut while the needle was still inserted, and then aspirated the wash liquid with the syringe. The aspirant was injected directly into a cryotube containing RNAlater. Facial skin samples were taken with sterile polyester swabs and collected in RNAlater. Diet of captive-bred birds The hawk and owl were fed with whole mice and day-old chicks. The turkey vultures received whole mice, chicks, rats, rabbits and guinea pigs, and horse and goat meat. Furthermore the flamingo diet was composed of commercial pellets containing maize, wheat and fishmeal manufactured by Kasper Faunafood, The Neatherlands and Nutrazu, UK, respectively. The parrot was fed on seeds fruits and vegetables. Finally, the seriema received a mix of day-old chicks, mice, mealworms, commercial dog food, commercial dried insect-mix, boiled eggs and a mix of vegetables. The faecal samples were sterile sampled and stored at −80 °C before DNA extraction. Mammalian DNA survey The DNA was extracted from facial swabs and hindgut aspirates with the FastDNA Spin kit for Soil (MP Biomedicals). 16S mammalian mtDNA was PCR amplified using mammalian primer set 16Smam1 5′-(CGGTTGGGGTGACCTCGGA)-3′ and 16Smam2 5′-(GCTGTTATCCCTAGGGTAACT)-3′ and a blocking oligo 16Smam_blkhum2 5′-(GCGACCTCGGAGCAGAACCC)-3′ (ref. 26 ). Both 16Smam1 and 16Smam2 were 5′-labelled with unique 8-nucleotide tags (with at least two differences between tags). All samples were amplified in duplicate with different tag combinations. This primer set is generic to mammals, excluding humans and related primates, and was specifically chosen to limit the chance of recovering a human signal that may derive from handling of vultures during collection and DNA extraction. PCR was performed using the enzyme Amplitaq Gold (Applied Biosystems, Foster City, CA) in 25 μl volumes that contained 1 mM MgCl 2 , 1 × buffer, 0.4 μM each primer, 0.1 mM mixed dNTPs, 0.1 μl Taq Gold and 1 μl purified DNA. In addition, 4.0 μM of a human blocking probe was added to each reaction to ensure as low an amplification of human DNA as possible [6] , [27] . PCR conditions were as follows: 95 °C for 5 min enzyme activation followed by 40 cycles of 95 °C for 12 s, 59 °C for 30 s and 70 °C for 25, and one cycle for final extension of 7 min at 70 °C. Post PCR, amplicons were visualized on 2% agarose gels stained with GelRed (Biotium, Hayward, CA). The PCR products were pooled in equimolar ratios and purified using Qiaquick PCR purification Kit (Qiagen, Valencia, CA) principally following the manufacturer’s guidelines, although including a 5 min incubation time at 37 °C before elution of the DNA. The purified PCR products were then build into indexed Illumina MiSeq libraries using the NEBNext Quick DNA Sample Prep Master Mix Set 2 (NEB, Ipswich, MA, USA). MiSeq sequencing was performed following the manufacturer’s protocol for paired-end reads, 150 bp settings. Illumina reads were trimmed using default settings in AdapterRemoval [28] , except using a minimal read length of 25 bp. After quality trimming, the paired sequences were merged using customized Perl scripts if the overlap was 100%. The trimmed and merged sequences were sorted in the sample-specific tag combinations using Geneious (Version 6.1.6 created by Biomatters). Sequences with tag-sequence errors were removed from further analysis. From each tag combination, OTUs with 97% similarity and a minimum number of 10 sequences were identified using Usearch [29] . OTUs were blasted and assigned to family using Geneious (Version 6.1.6 created by Biomatters). Only families present in both unique tag combinations from the same vulture sample were kept. 16S mammal sequences from facial swaps from two black vultures were excluded because only one tag combination amplified properly. All mammalian families observed are listed in Supplementary Table 1 . 16S rRNA gene amplicon sequencing We amplified the hypervariable region V3–V4 of the 16s rRNA gene using the 341F (5′-CCTAYGGGRBGCASCAG-3′) and 806R (5′-GGACTACNNGGGTATCTAAT-3′) primer and Phusion 540 l DNA Polymerase). The PCR reaction mix was composed of 5 μl 5 × Phusion buffer HF (7.5 mM MgCl 2 , Finnzymes, Finland), 0.5 μl 10 mM dNTPs, 1.25 μl 10 μM of each primer, 0.25 μl DNA polymerase (Hotstart Phusion 540 l, 1 unit per μl Finnzymes) and 1 μl template (same DNA extract that was used for the mammalian DNA survey). The reaction started with an initialization at 98 °C for 30 s, followed by 30 cycles of denaturation at 98 °C for 5 s, annealing at 56 °C for 20 s. and elongation at 72 °C for 10 s. The reaction was completed with a final elongation at 72 °C for 5 min. In the second PCR, the adaptors were attached to the amplicon library following the conditions of PCR I with only 15 cycles [30] . The 16S rRNA gene amplicon sequences were generated by one full plate of 454—Roche—FLX Titanium. The obtained observations were quality filtered, trimmed and split into the corresponding animal samples with the Qiime pipeline version 1.6.0 using the default settings [31] . Chimeras were removed by Uchime [32] and homopolymers truncated with AmpliconNoise [33] . On the basis of 650,697 trimmed sequences with the average length of 345bp of the wild vulture samples, OTUs were picked de novo and clustered at 97% sequence similarity (similar to species level). We generated 83,797 sequences of the seven zoo bird samples in the range of 10,932–13,716 reads per sample that were used for de novo OTU picking. The taxonomy was assigned using the Rdp classifier and Greengenes as reference database [34] , [35] . The rarefaction curves ( Supplementary Fig. 1 ) show the microbial richness (Chao1) in a given count of sequences. Both skin and hindgut curves reach asymptotes with fewer than 1,000 sequences. With an average of 4,544 sequences per sample, enough sequences were generated to characterize the microbial community of both skin and hindgut. Therefore we removed the difference in sequencing effort by randomly subsampling the OTU table at even sequencing depth of 4,544 observations. All further prokaryotic post analyses were based on the even OTU table. For statistical analysis, the even OTU table was transferred into the open source statistical program ‘R’ [36] . The normality of the raw data was evaluated with the Shapiro–Wilk test ( α =0.05). When variables were normally distributed, variation between two groups was investigated with the Welch’s t -test ( α =0.05), otherwise we used the nonparametric Wilcoxon Rank-Sum test ( α =0.05) to evaluate the differences in OTU alpha diversity between black and turkey vultures. Dissimilarities in OTU abundances between the samples were explained by the OTU count-based Bray–Curtis distance metric and examined by the analysis of similarity (ANOSIM). Microbial networks Bacteria that colonize the same environment potentially co-occur, sharing the same niche, or exclude each other while competing for the same resources. This relationship has been characterized in multiple investigations by generating the Spearman co-occurrence network on the basis of the relative OTU counts [37] . Positive pairwise correlations hypothetically indicate interactions such as symbiosis, mutualism or commensalism, whereas negative pairwise correlations potentially signal competition, mutual exclusion or parasitism. To reduce complexity, we omitted OTUs represented by fewer than 50 sequence observations. The network was generated using the CoNet plugin for Cytoscape on the basis of the nonparametric Spearman correlation coefficients with a minimal cutoff threshold of ρ =0.6 ( P ≪ 0.01, Bonferroni corrected) [38] , [39] . We present correlation data for OTUs that were detected in at least 50% of the gut samples ( n =13 for black vultures, n =11 for turkey vultures). The OTUs of the network of Fig. 3b represent 84% of the relative sequences of the black vulture samples, whereas the OTUs of Fig. 3c account for 73% of the relative sequences of the turkey vulture samples. The different interaction types are listed in Supplementary Table 9 . Hindgut metagenomic survey DNA from the hindgut of one turkey vulture was shotgun sequenced using the same DNA extract used to characterize prey composition and the microbial community. DNA in the extract was fragmented to 200–300 base pairs using Biorupter and the Illumina library was built by applying the NEB Blunt end Kit E6070. The library was amplified twice using different indexes in a 50 μl volume PCR mix containing 2 × Phusion High-Fidelity PCR Master Mix, 1 μM of Primer inPE1.0 (5′-AATGATACGGCGACCACCGAGATCTACACTCTTTCCCTACACGACGCTCTTCCGATCT)-3′, 20 nM of primer inPE2.0 (5′-GTGACTGGAGTTCAGACGTGTGCTCTTCCGATCT), 1 μM of an Illumina multiplex primer (5′-CAAGCAGAAGACGGCATACGAGATNNNNNNGTGACTGGAGTTC-3′, where the N stretch corresponds to a 6-nucleotide index tag) and 12 μl DNA extract. The PCR run was initialized at 98 °C for 30 s, and continued with 14 cycles of denaturation at 98 °C for 10 s, annealing at 65 °C for 30 s and elongation at 72 °C for 60 s. The reaction was finished with final step at 72 °C for 5 min. PCR products with the length of 325–425 bp were gel-cut and purified using QIAquick gel purification KIT and eluted in 22 μl EB buffer. The sequencing reaction followed the standard procedure of Illumina HiSeq2000 for paired-end reads. Raw reads were trimmed using the Cutadapt software with settings of minimum length 30 bp, minimum quality 30 and removal of all overrepresented sequence [40] . Cleaned raw reads were subject to an in-house chain-mapping using BWA-MEM as the mapping tool against bacterial genomes, vulture genome [41] , human genome and virus database in the given order [42] . The bacterial database consists of the 2,942 completely sequenced and draft genomes available in Genbank as of 22 January 2014, and the virus database consists of the complete Virus reference database from NCBI. All trimmed raw reads were additionally subject to BWA-MEM mapping against virulence genes [43] , and to the genomes of Meleagris gallopavo (Ensembl accession # GCA_000146605.1), Gallus gallus (Ensembl accession # GCA_000002315.2), Anas platyrhynchos (Ensembl accession # GCA_000355885.1), Equus caballus (Ensembl accession # GCA_000002305.1), Felis catus (Ensembl accession # GCA_000181335.2), Bos taurus (Ensembl accession # GCA_000003055.3), Sus scrofa (Ensembl accession # GCA_000003025.4), Rattus norvegicus (Ensembl accession # GCA_000001895.3), Ictidomys tridecemlineatus (Ensembl accession # GCA_000236235.1) and Oryctolagus cuniculus (Ensembl accession # GCA_000003625.1) as representatives of prey animals. All mappings were performed with paired-end data and the criteria for a positive hit were that both the reads should map with >80% of the read length in addition to the default settings in BWA-MEM. The majority of the data generated were assigned to vulture DNA (43.5%), unmapped reads (49%), bacteria (6.1%). Reads mapped against viruses were ≪ 0.01%. The sequences were submitted to the virulence factor database. The best hits are listed in Supplementary Table 7 . Accession codes: The microbiome sequence data from this study have been deposited in the NCBI Sequence Read Archive (SRA) with accession code SRP040754 . How to cite this article: Roggenbuck, M. et al. The microbiome of New World vultures. Nat. Commun. 5:5498 doi: 10.1038/ncomms6498 (2014).